LTD is a protein required for sorting light-harvesting chlorophyll-binding proteins to the chloroplast SRP pathway Higher plants require chloroplasts for essential functions in photosynthesis and other important physiological processes, such as sugar, lipid and amino-acid biosynthesis. Most chloroplast proteins are nuclear-encoded proteins that are synthesized in the cytosol as precursors, and imported into chloroplasts by protein translocases in the outer and inner chloroplast envelope. The imported chloroplast proteins are then translocated into or across the thylakoid membrane by four distinct pathways. However, the mechanisms by which the imported nuclear-encoded proteins are delivered to these pathways remain largely unknown. Here we show that an Arabidopsis ankyrin protein, LTD (mutation of which causes the light-harvesting chlorophyll-binding protein translocation defect), is localized in the chloroplast and using yeast two-hybrid screens demonstrate that LTD interacts with both proteins from the signal recognition particle (SRP) pathway and the inner chloroplast envelope. Our study shows that LTD is essential for the import of light-harvesting chlorophyll-binding proteins and subsequent routing of these proteins to the chloroplast SRP-dependent pathway. Correct and efficient targeting and translocation of proteins from their sites of synthesis into or across a membrane to their functional compartments is a fundamental process [1] , [2] . Chloroplasts contain about 3,000 proteins, but only 50–200 of them are encoded for in the plastid genome. Nuclear-encoded proteins are synthesized in the cytosol and post-translationally translocated across the chloroplast envelopes [1] , [2] , [3] , [4] , [5] , [6] . The protein import complexes located on the outer and inner envelope membranes are termed as TOC (translocon at the outer envelop membrane of chloroplast) and TIC (translocon at the inner envelop membrane of chloroplast) complexes, respectively [1] , [2] , [5] , [6] . The Toc159, Toc75 and Toc34 proteins form the core TOC complex and are involved in protein transport across the outer envelope [6] , [7] , [8] . Tic110, Tic20 and Tic21 have been suggested to function as the protein translocation channel of the inner envelope [1] , [2] , [7] , [8] . Several stromal proteins, including chaperones, proteases and redox regulators, are also involved in the import process [6] , [9] , [10] . The stromal domain of Tic110 and Hip/Hop domain of Tic40 may function as scaffolds that tether stromal chaperones, including Hsp93 and Hsp70, which facilitate protein translocation across the inner membrane [2] , [6] , [11] . After translocation across the envelope, imported proteins are inserted into or transported across the thylakoid membrane through one of four mechanistically distinct pathways, which are classified on the basis of their energy and stromal factor requirements [3] , [4] : the Sec-dependent pathway, the twin-arginine translocation (Tat) pathway, the chloroplast signal recognition particle (cpSRP) pathway and the spontaneous insertion pathway. The Sec pathway requires a translocation ATPase, SecA, and the translocation channel consisting of SecY and SecE, and is involved in transport of several lumenal proteins including plastocyanin and 33-kDa protein of the oxygen-evolving complex (OE33) (ref. 12 ). The cpSRP pathway uses GTP, cpSRP54, cpSRP43, cpFtsY and Alb3 to target the abundant light-harvesting chlorophyll a/b-binding proteins (LHCP) to the thylakoid membrane [13] , [14] . The Tat pathway uses a trans -thylakoid pH gradient as its sole energy source, and Tha4, Hcf106 and TatC may form a complex for the transport of a subset of lumen proteins, such as the 17- and 23-kDa proteins of the oxygen-evolving complex (OE17 and OE23) (ref. 4 ). The 'spontaneous' pathway does not seem to require soluble factors or energy and is the mode of insertion of CFoII, PSII-W, PSII-X and ELIP into the membrane [3] , [4] . Although these pathways can be distinguished by their protein factors and energy requirements, how imported chloroplast proteins are sorted to these distinct pathways is still unknown. LHCP form a soluble transit complex with cpSRP, which consists of cpSRP54 and cpSRP43, after import into the chloroplast [15] , [16] , [17] . The ankyrin domain of cpSRP43 interacts with a conserved L18 region between the second and third transmembrane domains of LHCP [18] , [19] . Targeting of LHCP to the membrane also requires the chloroplast SRP receptor homologue cpFtsY and GTP [20] . In the presence of GTP, cpFtsY interacts with cpSRP to promote GTP binding of both cpSRP54 and cpFtsY, which contain GTPase domains. On GTP hydrolysis, cpSRP is released from the membrane, and insertion of LHCP into the thylakoid membrane is mediated by the integral membrane protein Alb3 (refs 21 , 22 ). Besides the above typical cpSRP pathway, some LHCP might be able to bypass cpSRP54 and cpFtsY, and undergo cpFtsY-independent targeting to the membrane by cpSRP43 and Alb3 (refs 23 , 24 ). Previous studies on the mechanisms of LHCP targeting to chloroplasts have largely focused on how LHCP are inserted into the thylakoid membrane by the cpSRP pathway [13] . However, the mechanisms of how LHCP are delivered to the cpSRP pathway during or after translocation across the envelope remain largely unknown. In this study, we characterized the LHCP translocation defect ( ltd ) mutant and found that l ight-harvesting chlorophyll-binding protein t ranslocation d efect (LTD) is involved in both facilitating LHCP translocation across the inner envelope and subsequently delivering them to the cpSRP pathway. The ltd mutant displays defects in LHCP biogenesis The At1g50900 gene encodes a protein of 175 amino acids, with a putative chloroplast transit peptide of 68 amino acids in its amino (N) terminus ( Supplementary Fig. S1 ). This protein is predicated to contain one ankyrin repeat between residues 117 and 149 ( Supplementary Fig. S1 ). At1g50900 was designated LTD because its mutation leads to LHCP translocation defect. Homologues of At1g50900 were found in higher plants, moss and green algae ( Supplementary Fig. S1 ). The At1g50900 gene contains two exons and one intron, and the mutant ltd carries a T-DNA insertion at the second exon ( Supplementary Fig. S2 ). The ltd seedlings were not able to grow photoautotrophically in soil, but could be maintained on sucrose-supplemented medium. However, they did not develop fertile flowers. The ltd mutant had yellow leaves and showed retarded growth compared with wild-type plants ( Fig. 1a ). The total chlorophyll contents in ltd were 5% of that of wild type, and the chlorophyll a/b ratio was 7.1 in ltd mutants, compared with 3.4 in the wild type ( Fig. 1b ). Because LHCP are the only proteins that bind chlorophyll b [25] , the increased chlorophyll a/b ratio suggests that the LTD mutation affects LHCP accumulation but does not rule out other effects. Transmission electron microscopy analysis showed that wild-type chloroplasts contained well-developed thylakoids and substantial granal stacks ( Fig. 1c ). However, grana stacking was impaired in ltd chloroplasts, which further suggests that the LTD mutation affects LHCP biogenesis [26] , [27] . 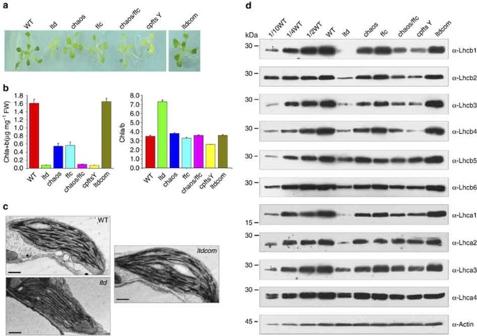Figure 1: Theltdmutant displays defects in the accumulation of LHCP and chloroplast development. (a) Phenotypes of the wild-type (WT),ltd,chaos,ffc,cpftsy,chaos/ffcandltdcomplemented with full-length LTD (ltdcom) plants grown on MS plates containing 3% sucrose for 3 weeks. (b) Chlorophyll contents and chl a/b ratios of 3-week-old WT,ltd, chaos, ffc, chaos/ffc,cpftsYandltdcomseedlings. FW, fresh weight. Data are the means±s.e. (n=7). (c) Transmission electron microscopic images of the chloroplast ultrastructure in WT,ltdandltdcomleaf sections from the plants shown ina. Scale bar, 1 μm. (d) Immunoblot analysis of LHCI and LHCII in total leaf proteins extracted from 3-week-old WT,ltd, chaos, ffc, cpftsY,chaos/ffcandltdcomplants. Actin served as controls to normalize protein levels. Similar results were obtained in two additional independent experiments. Figure 1: The ltd mutant displays defects in the accumulation of LHCP and chloroplast development. ( a ) Phenotypes of the wild-type (WT), ltd , chaos , ffc , cpftsy , chaos/ffc and ltd complemented with full-length LTD ( ltdcom ) plants grown on MS plates containing 3% sucrose for 3 weeks. ( b ) Chlorophyll contents and chl a/b ratios of 3-week-old WT, ltd, chaos, ffc, chaos/ffc , cpftsY and ltdcom seedlings. FW, fresh weight. Data are the means±s.e. ( n =7). ( c ) Transmission electron microscopic images of the chloroplast ultrastructure in WT, ltd and ltdcom leaf sections from the plants shown in a . Scale bar, 1 μm. ( d ) Immunoblot analysis of LHCI and LHCII in total leaf proteins extracted from 3-week-old WT, ltd, chaos, ffc, cpftsY , chaos/ffc and ltdcom plants. Actin served as controls to normalize protein levels. Similar results were obtained in two additional independent experiments. Full size image To elucidate the LTD function, we compared the effects of LTD inactivation on LHCP biogenesis with Arabidopsis mutants known to have defects in LHCP biogenesis ( chaos , which lacks cpSRP43; ffc , which lacks cpSRP54; and cpftsY , which lacks cpFtsY) [16] , [23] , [28] ( Fig. 1d ). Immunoblot analysis showed that LHCP in ltd were more severely reduced than in mutants that lack cpSRP pathway components. In particular, Lhcb1, Lhcb2, Lhca1 and Lhca2 were reduced to <5% of wild-type levels. Tic110, Tic40, cpHsp93, cpHsp70, cpSRP43, cpSRP54 and cpFtsY accumulated rather normally or were increased in ltd ( Supplementary Fig. S3a ), which suggests that the reduction in LHCP levels was not the result of secondary effects of the LTD mutation on other import components. The levels of chloroplast proteins were also examined in ltd using specific antibodies ( Supplementary Fig. S3a ). The PSI and PSII core subunits PsaA/B, D2 and CP47 were reduced to about 50% of wild-type levels, whereas the levels of OE33, Cytf of Cytb 6 /f and the β-subunit of ATP synthase were unchanged compared with wild type. A previous report suggested that depletion of LHCP might result in impaired stability of photosynthetic proteins [29] . Pulse labelling for 20 min followed by a chase with unlabelled methionine in the presence of cycloheximide, which blocks the synthesis of nuclear-encoded proteins, showed that the turnover rates of the PSI and PSII subunits (PsaA/B, CP47, CP43, D1 and D2) were higher in ltd than in wild-type plants ( Supplementary Fig. S3b ). Thus, the reduced levels of the PSI and PSII core proteins are caused by reduced stability in ltd . Cellular localization of LTD To characterize the LTD function, we first determined its subcellular localization. The LTD-green fluorescent protein (GFP) fusion protein was transiently expressed in protoplasts [30] , and GFP fluorescence exclusively co-localized with chloroplastic chlorophyll ( Fig. 2a ). This localization was similar to that of GFP fused to the transit peptide of LPA66 (ref. 31 ). GFP fusion proteins with the targeting signals of fibrillarin [32] and FRO1 (ref. 33 ) of Arabidopsis were located specifically in the nucleus and mitochondria, respectively ( Fig. 2a ). These results confirm that LTD is indeed localized to the chloroplast. 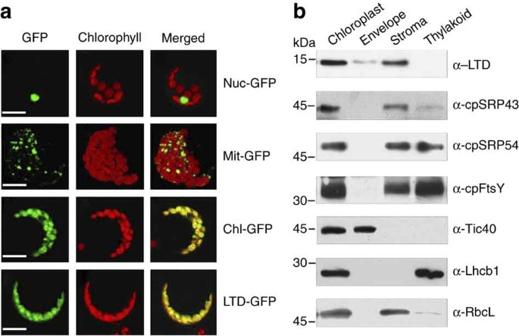Figure 2: Localization of LTD. (a) Subcellular localization of the LTD protein by GFP fluorescence. Green indicates GFP, red shows chloroplast autofluorescence and yellow shows co-localization in the merged images. The constructs used for transformation are indicated at the right: Nuc-GFP, control nuclear localization signal of fibrillarin; Mit-GFP, control mitochondrial localization signal of FRO1; Chl-GFP, control chloroplast localization signal of LPA66-GFP fusion protein; LTD-GFP, signal from the LTD-GFP fusion protein. Scale bars, 5 μm. (b) Immunolocalization analysis of LTD. The chloroplast, envelope, stromal and thylakoid fractions were subjected to immunoblot analysis with specific antisera against LTD, cpSRP43, cpSRP54, cpFtsY, Tic40, Lhcb1 and RbcL (ribulose-1,5-bisphosphate carboxylase/oxygenase large subunit). Equal amounts of protein (10 μg) were loaded in each lane. Similar results (a,b) were obtained in two additional independent experiments. Figure 2: Localization of LTD. ( a ) Subcellular localization of the LTD protein by GFP fluorescence. Green indicates GFP, red shows chloroplast autofluorescence and yellow shows co-localization in the merged images. The constructs used for transformation are indicated at the right: Nuc-GFP, control nuclear localization signal of fibrillarin; Mit-GFP, control mitochondrial localization signal of FRO1; Chl-GFP, control chloroplast localization signal of LPA66-GFP fusion protein; LTD-GFP, signal from the LTD-GFP fusion protein. Scale bars, 5 μm. ( b ) Immunolocalization analysis of LTD. The chloroplast, envelope, stromal and thylakoid fractions were subjected to immunoblot analysis with specific antisera against LTD, cpSRP43, cpSRP54, cpFtsY, Tic40, Lhcb1 and RbcL (ribulose-1,5-bisphosphate carboxylase/oxygenase large subunit). Equal amounts of protein (10 μg) were loaded in each lane. Similar results ( a , b ) were obtained in two additional independent experiments. Full size image To determine the LTD localization within chloroplasts, intact chloroplasts were isolated and fractionated, and the proteins were separated by SDS–polyacrylamide gel electrophoresis (PAGE) followed by immunoblot analysis ( Fig. 2b ). Most of the LTD protein was detected in the stromal fractions, and a small amount was found in the envelope factions, whereas none was detected in the thylakoid fractions ( Fig. 2b ). cpSRP43, cpSRP54 and cpFtsY were detected both in the chloroplast stromal and thylakoid fractions, whereas most of the cpSRP43 protein was found in the stromal fractions. cpSRP54 was distributed almost equally between the stroma and thylakoids, and cpFtsY was mainly associated with the thylakoid membrane ( Fig. 2b ), which is consistent with previous reports [16] , [23] , [34] , [35] . LTD interacts with cpSRP43 and TIC components To further investigate the LTD function, we used a protein overlay assay to detect its interaction proteins in the stroma ( Fig. 3a ). 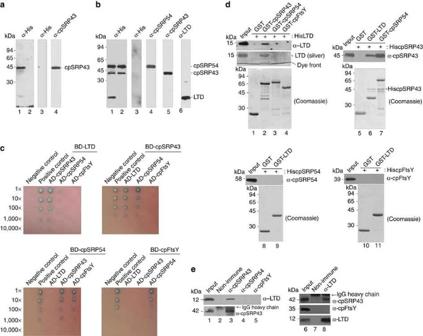Figure 3: LTD interacts with cpSRP43. (a) Protein overlay analysis of LTD protein interactions. Overlay of the His-tagged LTD protein on the blots of wild-type (line 1, 3, 4) orchaosmutant (lane 2) stromal proteins (30 μg per gel) was followed by immunodetection with anti-His antibody or directly immunolabeled with antibody indicated on the top. (b) Protein overlay analysis of cpSRP43 protein interactions. Overlay of the His-tagged cpSRP43 protein on wild-type (lane 1, 3, 4, 5, 6) andltdmutant (line 2) stromal proteins (30 μg per gel) was followed by immunoblot analysis with an anti-His antibody (lanes 1–2) or directly immunolabeled with antibody indicated on the top. (c) Yeast two-hybrid analyses of the interactions between LTD, cpSRP43, cpSRP54 and cpFtsY. Plasmid construction and yeast two-hybrid analyses were performed as described in the Methods. (d) Pull-down assay. Full-length His-tagged LTD was used as the prey, and full-length GST-tagged cpSRP43, cpSRP54 and cpFtsY were used as bait, respectively (lane 2–4); full-length GST-tagged LTD was used as the bait, and full-length His-tagged cpSRP43, cpSRP54 and cpFtsY were used as prey, (lanes 6, 9, 10) respectively; full-length His-tagged cpSRP43 was used as the prey, and GST-tagged cpSRP54 were used as bait (lane 8). The purified recombinant proteins were bound to glutathione-agarose beads, and the bound proteins were eluted and analysed by immunoblot or staining. The positions of LTD in silver-stained gel and cpSRP43 in Coomassie-stained gel were indicated on the right. Input, 4% of the prey protein. (e) Co-immunoprecipitation analysis of the interaction between cpSRP43 and LTD.Arabidopsischloroplast stromal proteins were first immunoprecipitated with non-immune serum (lanes 2 and 7) or antibodies against cpSRP43 (lane 3), cpSRP54 (lane 4), cpFtsY (lane 5) or LTD (lane 8) then analysed by immunoblot with antibodies indicated on the right. Input (lanes 1 and 6) indicates that 10 μg stromal proteins were loaded on the gel. The positions of the IgG heavy chain are indicated with arrows. As shown in Figure 3a , LTD bound to cpSRP43; however, no signal was detected when the membrane was blotted either with chaos stromal protein or with wild-type stromal proteins in the absence of LTD ( Fig. 3a ). Overlays performed with the wild-type stromal proteins revealed that cpSRP43 interacted with cpSRP54, cpSRP43 and LTD ( Fig. 3b ). A parallel set of protein overlay experiments using ltd stromal proteins showed the interaction between cpSRP54 and cpSRP43, which is consistent with the formation of a stable cpSRP43 and cpSRP54 heterodimer [19] , [36] . However, cpSRP43 has also been suggested to be a dimer through gel filtration and chemical cross-linking experiments [20] . Yeast two-hybrid analysis revealed that the third and fourth ankyrin repeats are responsible for the dimerization [37] . Equilibrium ultracentrifugation analysis showed that it is a monomer; however, a cpSRP43 mutant protein lacking the carboxy (C)-terminal chromodomains was able to form a stable dimer [36] . These together with our protein overlay results suggest a potential dimerization of cpSRP43 (ref. 14 ). Figure 3: LTD interacts with cpSRP43. ( a ) Protein overlay analysis of LTD protein interactions. Overlay of the His-tagged LTD protein on the blots of wild-type (line 1, 3, 4) or chaos mutant (lane 2) stromal proteins (30 μg per gel) was followed by immunodetection with anti-His antibody or directly immunolabeled with antibody indicated on the top. ( b ) Protein overlay analysis of cpSRP43 protein interactions. Overlay of the His-tagged cpSRP43 protein on wild-type (lane 1, 3, 4, 5, 6) and ltd mutant (line 2) stromal proteins (30 μg per gel) was followed by immunoblot analysis with an anti-His antibody (lanes 1–2) or directly immunolabeled with antibody indicated on the top. ( c ) Yeast two-hybrid analyses of the interactions between LTD, cpSRP43, cpSRP54 and cpFtsY. Plasmid construction and yeast two-hybrid analyses were performed as described in the Methods. ( d ) Pull-down assay. Full-length His-tagged LTD was used as the prey, and full-length GST-tagged cpSRP43, cpSRP54 and cpFtsY were used as bait, respectively (lane 2–4); full-length GST-tagged LTD was used as the bait, and full-length His-tagged cpSRP43, cpSRP54 and cpFtsY were used as prey, (lanes 6, 9, 10) respectively; full-length His-tagged cpSRP43 was used as the prey, and GST-tagged cpSRP54 were used as bait (lane 8). The purified recombinant proteins were bound to glutathione-agarose beads, and the bound proteins were eluted and analysed by immunoblot or staining. The positions of LTD in silver-stained gel and cpSRP43 in Coomassie-stained gel were indicated on the right. Input, 4% of the prey protein. ( e ) Co-immunoprecipitation analysis of the interaction between cpSRP43 and LTD. Arabidopsis chloroplast stromal proteins were first immunoprecipitated with non-immune serum (lanes 2 and 7) or antibodies against cpSRP43 (lane 3), cpSRP54 (lane 4), cpFtsY (lane 5) or LTD (lane 8) then analysed by immunoblot with antibodies indicated on the right. Input (lanes 1 and 6) indicates that 10 μg stromal proteins were loaded on the gel. The positions of the IgG heavy chain are indicated with arrows. Full size image To examine whether LTD interacts with other proteins related to the cpSRP pathway, yeast two-hybrid assays were performed ( Fig. 3c ). As shown in Figure 3c , LTD interacted with cpSRP43 but not with cpSRP54 and cpFtsY. Pull-down assays provided further support for the interaction between cpSRP43 and LTD ( Fig. 3d ). Co-immunoprecipitation analysis revealed that the interaction between LTD and cpSRP43 also occurs in vivo , although the interaction appeared weak ( Fig. 3e ). Because LTD only interacts with cpSRP43 and not cpSRP54, it is possible that LTD is not a component of the transit complex. To test this, chloroplast stromal proteins were separated by sucrose gradient sedimentation and analysed by immunoblot using specific antibodies ( Supplementary Fig. S4 ). Immunoblot analysis showed that LTD did not co-migrate with cpSRP43 and cpSRP54. Because LTD was also found to be associated with the envelope membrane, we next studied its interactions with inner envelope proteins. 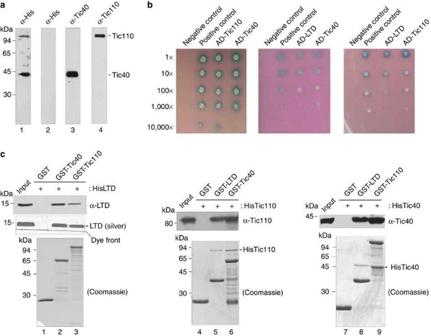Figure 4: LTD interacts with the TIC complex. (a) Protein overlay analysis of the LTD interactions with Tic40 and Tic110. Overlay of the recombinant His-tagged LTD protein on wild-type inner envelope proteins (20 μg per gel) was followed by immunodetection with anti-His antibody (lane 1) or directly immunodetected with antibody indicated on the top. (b) Yeast two-hybrid analyses of interactions between LTD, Tic40 and Tic110. Full-length LTD, full-length Tic40 and the C-terminal part of the Tic110 stromal domain (amino acids 385–1,016) were fused to the GAL4 DNA-binding domain (BD; left BD-LTD, middle BD-Tic110, and right BD-Tic40) and the GAL4 activation domain (AD). (c) Protein pull-down assays. Lanes 1–3: full-length His-tagged LTD was used as the prey, and GST, full-length GST-tagged Tic40, and C-terminal parts of Tic110 stromal domain (amino acids 385–1,016) were used as bait, respectively. Lanes 4–6: C-terminal part of the Tic110 stromal domain (amino acids 385–1,016) fused to His-tag was used as the prey, and GST, full-length GST-tagged LTD and Tic40 were used as bait, respectively. Lanes 7–9: C-terminal part of the Tic40 stromal domain (amino acids 128–447) fused with His-tag was used as the prey, and GST, full-length GST-tagged LTD and Tic110 were used as bait, respectively. The purified recombinant proteins were bound to glutathione-agarose beads, eluted and analysed by 15% SDS–PAGE followed by immunoblot analysis using the antibodies indicated on the right. Images of silver-stained and Coomassie-stained gels are shown below the immunoblot. Input, 4% of the prey protein. As shown in Figure 4a , LTD bound to Tic110 and Tic40. Furthermore, yeast two-hybrid and pull-down assays provided further evidence that LTD indeed interacts with Tic110 and Tic40 ( Fig. 4b,c ). Figure 4: LTD interacts with the TIC complex. ( a ) Protein overlay analysis of the LTD interactions with Tic40 and Tic110. Overlay of the recombinant His-tagged LTD protein on wild-type inner envelope proteins (20 μg per gel) was followed by immunodetection with anti-His antibody (lane 1) or directly immunodetected with antibody indicated on the top. ( b ) Yeast two-hybrid analyses of interactions between LTD, Tic40 and Tic110. Full-length LTD, full-length Tic40 and the C-terminal part of the Tic110 stromal domain (amino acids 385–1,016) were fused to the GAL4 DNA-binding domain (BD; left BD-LTD, middle BD-Tic110, and right BD-Tic40) and the GAL4 activation domain (AD). ( c ) Protein pull-down assays. Lanes 1–3: full-length His-tagged LTD was used as the prey, and GST, full-length GST-tagged Tic40, and C-terminal parts of Tic110 stromal domain (amino acids 385–1,016) were used as bait, respectively. Lanes 4–6: C-terminal part of the Tic110 stromal domain (amino acids 385–1,016) fused to His-tag was used as the prey, and GST, full-length GST-tagged LTD and Tic40 were used as bait, respectively. Lanes 7–9: C-terminal part of the Tic40 stromal domain (amino acids 128–447) fused with His-tag was used as the prey, and GST, full-length GST-tagged LTD and Tic110 were used as bait, respectively. The purified recombinant proteins were bound to glutathione-agarose beads, eluted and analysed by 15% SDS–PAGE followed by immunoblot analysis using the antibodies indicated on the right. Images of silver-stained and Coomassie-stained gels are shown below the immunoblot. Input, 4% of the prey protein. Full size image LTD interacts with both precursor and mature LHCP The interaction of LTD with Tic110 and Tic40 suggests that LTD could interact with pLHCP during import. To test this possibility, in vitro -translated [ 35 S]pLHCP were incubated with isolated chloroplasts under normal import conditions. After incubation for 5 and 20 min, both pLHCP and mature LHCP (mLHCP) could be precipitated with the anti-LTD antibody under nondenaturing conditions, but the pLHCP/mLHCP ratio was reduced after 20 min ( Fig. 5a ). In comparison, the cpSRP43 antibody only precipitated mLHCP under these conditions. After a 40 min incubation, neither LTD nor cpSRP43 antibody could precipitate LHCP. 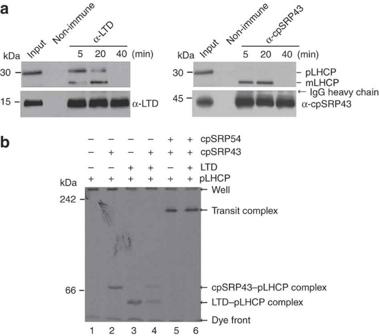Figure 5: LTD interacts with LHCP. (a) LTD is associated with importing pLHCP. Chloroplasts were incubated with [35S]pLHCP under import conditions for 5, 20 or 40 min; reisolated; solubilized with 1% docecyl β-Dmaltoside and subjected to immunoprecipitation with non-immune serum or antibodies against LTD and cpSRP43. The immunoprecipitates were analysed by 15% SDS–PAGE or 10% Tricine-SDS–PAGE gels (for the immunoblot analysis of LTD) and Coomassie staining, autoradiography (upper panel) or immunoblot analysis with the indicated antibodies (lower panel). The position of the IgG heavy chain is indicated with an arrow. Input, 1% of the solubilized chloroplast supernatant used for immunoprecipitation. (b) LTD forms a soluble complex with pLHCP. Synthesized pLHCP were incubated with purified recombinant LTD (200 ng), cpSRP54 (200 ng) and cpSRP43 (400 ng) as described in the Methods. After incubation, the samples were separated on 6–12% nondenaturing gels and visualized by autoradiography. The transit complex (lanes 5 and 6), cpSRP43–pLHCP (lanes 2 and 4) and LTD–pLHCP (lanes 3 and 4) complexes are indicated with arrows. pLHCP alone are used as a control (lane 1). Figure 5: LTD interacts with LHCP. ( a ) LTD is associated with importing pLHCP. Chloroplasts were incubated with [ 35 S]pLHCP under import conditions for 5, 20 or 40 min; reisolated; solubilized with 1% docecyl β- D maltoside and subjected to immunoprecipitation with non-immune serum or antibodies against LTD and cpSRP43. The immunoprecipitates were analysed by 15% SDS–PAGE or 10% Tricine-SDS–PAGE gels (for the immunoblot analysis of LTD) and Coomassie staining, autoradiography (upper panel) or immunoblot analysis with the indicated antibodies (lower panel). The position of the IgG heavy chain is indicated with an arrow. Input, 1% of the solubilized chloroplast supernatant used for immunoprecipitation. ( b ) LTD forms a soluble complex with pLHCP. Synthesized pLHCP were incubated with purified recombinant LTD (200 ng), cpSRP54 (200 ng) and cpSRP43 (400 ng) as described in the Methods. After incubation, the samples were separated on 6–12% nondenaturing gels and visualized by autoradiography. The transit complex (lanes 5 and 6), cpSRP43–pLHCP (lanes 2 and 4) and LTD–pLHCP (lanes 3 and 4) complexes are indicated with arrows. pLHCP alone are used as a control (lane 1). Full size image To further investigate the LTD function in LHCP targeting, we tested the abilities of LTD, cpSRP43 and cpSRP54 to form a protein complex with in vitro- translated [ 35 S]pLHCP ( Fig. 5b ). As expected, the transit complex was formed when recombinant cpSRP54 and cpSRP43 were incubated with [ 35 S]pLHCP [18] , [36] . Incubation of [ 35 S]pLHCP with cpSRP43 resulted in the formation of a cpSRP43–pLHCP complex, which is consistent with previous reports that cpSRP43 alone prevents aggregation of LHCP by complex formation [38] . As shown in Figure 5b , a LTD–pLHCP complex was also formed when [ 35 S]pLHCP was mixed with LTD. In addition, incubation of pLHCP with LTD and cpSRP43 led to the formation of a LTD–pLHCP complex and a cpSRP43–pLHCP complex. However, when [ 35 S]pLHCP were incubated with cpSRP43, cpSRP54 and LTD, a new complex was observed to form, as the LTD–pLHCP complex disappeared ( Fig. 5b ). Because this complex co-migrated with the transit complex containing pLHCP, cpSRP43 and cpSRP54, it is possible that LTD is not a component of the transit complex. LTD recognizes a specific region in LHCP As cpSRP43 specifically recognizes the L18 region in LHCP [18] , [19] , we next investigated whether LTD also recognizes a specific region in LHCP. An alignment of the amino-acid sequences of LHCP (Lhcb1-6 and Lhca1-4) revealed several strictly conserved amino-acid regions ( Supplementary Fig. S5 ). To identify the amino-acid sequence that mediates the interaction between LTD and LHCP, five contiguous conserved segments in pLHCP, corresponding to amino acids 51–90, 91–135, 163–206, 207–255 and 228–267 (indicated by red arrows in Supplementary Fig. S5 ), were used in Gal4-based yeast two-hybrid and pull-down assays ( Fig. 6 ). 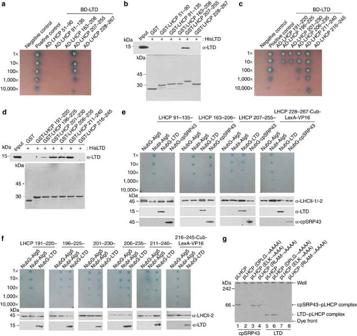Figure 6: LTD binds to the T14 region of LHCP. (a) Gal4-based yeast two-hybrid analyses of the interaction between LTD and various deletion mutants of LHCP (Lhcb1 amino acids 51–90, 91–135, 163–206, 207–255 and 228–267). (b) Protein pull-down assays of the LTD interaction with various deletion mutants of LHCP. GST-tagged various deletion mutants of LHCP were used as bait, which were indicated on the top. An image of the Coomassie-stained gel is shown below the immunoblot. Input, 4% of prey protein. (c) Gal4-based yeast two-hybrid analyses of the interaction between LTD and various deletion mutants of LHCP (Lhcb1 amino acids 191–220, 196–225, 201–230, 206–235, 211–240 or 216–245). (d) Protein pull-down assays of the interaction between LTD and various deletion mutants of LHCP (Lhcb1 amino acids 191–220, 196–225, 201–230, 206–235, 211–240 or 216–245). An image of the Coomassie-stained gel is shown below the immunoblot. Input, 4% of prey protein. (e) Split ubiquitin-based yeast two-hybrid analyses. Full-length LTD or cpSRP43 fused to the NubG fragment of the pDSLNx vector was used as the prey, and various deletion mutants of LHCP (Lhcb1 amino acids 91–135, 163–206, 207–255, 228–267) fused to Cub-LexA-VP16 fragment of PCCW vector were used as bait. Immunoblot analysis of total protein extracts from the NMY32-transformed yeast cells were performed with anti-LTD, anti-cpSRP43, anti-LHCII-1 (against amino acids 24–152 of Lhcb1) and anti-LHCII-2 (against amino acids 175–245 of Lhcb1) antibodies (bottom). (f) Split ubiquitin-based yeast two-hybrid analyses of the interaction between LTD and various deletion mutants of LHCP (Lhcb1 amino acids 191–220, 196–225, 201–230, 206–235, 211–240 or 216–245). Immunoblot analysis of total protein extracts from the NMY32-transformed yeast cells were indicated on the bottom. (g) The effects of the T14 mutation on LTD interaction with pLHCP. The synthesized pLHCP or pLHCP substitution mutant proteins were incubated with purified recombinant cpSRP43 (lanes 1–4; 400 ng) or LTD (lanes 5–8; 200 ng) proteins as described in the Methods. After incubation, the samples were assayed for the formation of complexes on 6–12% nondenaturing gels and visualized by autoradiography. The cpSRP43–pLHCP and LTD–pLHCP complexes are indicated with arrows. As shown in Figure 6a,b , LTD only interacted with pLHCP 207−255 and not with other segments. Figure 6: LTD binds to the T14 region of LHCP. ( a ) Gal4-based yeast two-hybrid analyses of the interaction between LTD and various deletion mutants of LHCP (Lhcb1 amino acids 51–90, 91–135, 163–206, 207–255 and 228–267). ( b ) Protein pull-down assays of the LTD interaction with various deletion mutants of LHCP. GST-tagged various deletion mutants of LHCP were used as bait, which were indicated on the top. An image of the Coomassie-stained gel is shown below the immunoblot. Input, 4% of prey protein. ( c ) Gal4-based yeast two-hybrid analyses of the interaction between LTD and various deletion mutants of LHCP (Lhcb1 amino acids 191–220, 196–225, 201–230, 206–235, 211–240 or 216–245). ( d ) Protein pull-down assays of the interaction between LTD and various deletion mutants of LHCP (Lhcb1 amino acids 191–220, 196–225, 201–230, 206–235, 211–240 or 216–245). An image of the Coomassie-stained gel is shown below the immunoblot. Input, 4% of prey protein. ( e ) Split ubiquitin-based yeast two-hybrid analyses. Full-length LTD or cpSRP43 fused to the NubG fragment of the pDSLNx vector was used as the prey, and various deletion mutants of LHCP (Lhcb1 amino acids 91–135, 163–206, 207–255, 228–267) fused to Cub-LexA-VP16 fragment of PCCW vector were used as bait. Immunoblot analysis of total protein extracts from the NMY32-transformed yeast cells were performed with anti-LTD, anti-cpSRP43, anti-LHCII-1 (against amino acids 24–152 of Lhcb1) and anti-LHCII-2 (against amino acids 175–245 of Lhcb1) antibodies (bottom). ( f ) Split ubiquitin-based yeast two-hybrid analyses of the interaction between LTD and various deletion mutants of LHCP (Lhcb1 amino acids 191–220, 196–225, 201–230, 206–235, 211–240 or 216–245). Immunoblot analysis of total protein extracts from the NMY32-transformed yeast cells were indicated on the bottom. ( g ) The effects of the T14 mutation on LTD interaction with pLHCP. The synthesized pLHCP or pLHCP substitution mutant proteins were incubated with purified recombinant cpSRP43 (lanes 1–4; 400 ng) or LTD (lanes 5–8; 200 ng) proteins as described in the Methods. After incubation, the samples were assayed for the formation of complexes on 6–12% nondenaturing gels and visualized by autoradiography. The cpSRP43–pLHCP and LTD–pLHCP complexes are indicated with arrows. Full size image To further narrow down which LHCP regions are involved in the LTD-mediated protein interaction, serial overlapping 30 amino-acid segments of LHCP were fused to the GAL4 activation domain or a GST tag for yeast two-hybrid and pull-down assays, respectively ( Fig. 6c,d ). LTD interacted with segments of pLHCP that corresponded to amino acids 196–225, 201–230, 206–235, and 211–240, but not with either pLHCP 191−220 or pLHCP 216−245 . We next used a split ubiquitin-based two-hybrid system to further test the interaction of LTD with the pLHCP segments in the transmembrane regions (amino acids 91–135, 163–206, 207–255 and 228–255). As shown in Figure 6e,f , similar results were obtained using this system. As expected, cpSRP43 interacted with the pLHCP 163−206 region, which contains the L18 region [18] , [19] ( Fig. 6e ). These results suggested that the 14 amino-acid sequence, T14 (located at the beginning of the third transmembrane domain), is an essential element for the LTD-mediated protein interaction (amino acids 211–224 of pLHCP; red box in Supplementary Fig. S5 ). The amino-acid sequences ELK and RLAM, similar to DPLG motif in L18, are the most conserved in T14 ( Supplementary Fig. S5 ). We therefore generated three substitution mutants, pLHCP-DPLG, pLHCP-ELK and pLHCP-RLAM, which had Ala substitutions in the L18 or T14 regions. Incubation of pLHCP-ELK or pLHCP-RLAM with LTD did not yield the pLHCP–LTD complex, whereas these pLHCP substitution mutants could form complexes with cpSRP43 ( Fig. 6g ). However, pLHCP-DPLG could form complexes with LTD but not with cpSRP43. These results further confirmed the essential function of T14 in the protein interactions of LTD. T14 is essential for pLHCP translocation across the envelope To clarify the function of this specific region in protein translocation, a synthetic peptide corresponding to T14 fused to the transit peptide of pLHCP (TpT14) was used to compete with pLHCP during protein translocation ( Fig. 7a,b ). The specific cpSRP43-binding domain L18 fused to the transit peptide of pLHCP was used as the control (TpL18). 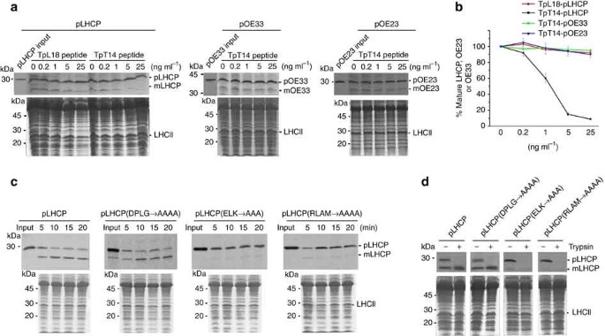Figure 7: T14 is important for pLHCP protein translocation across the inner membrane. (a) A synthetic peptide corresponding to T14 competes with pLHCP for translocation across the envelope. Chloroplasts were isolated from 3-week-oldArabidopsisplants and incubated with [35S]pLHCP, [35S]pOE33 or [35S]pOE23 for 10 min in the presence of increasing concentrations of TPT14 or TPL18 peptide (as described in the Methods). After incubation, the intact chloroplasts were reisolated, and the chloroplast proteins were separated on 15% SDS–PAGE gels and visualized by autoradiography. (b) Quantification of imported mature [35S]LHCP, [35S]OE33 or [35S]OE23 relative to the amount of endogenous LHCP resolved by SDS–PAGE. The amount of mature [35S]LHCP, [35S]OE33 or [35S]OE23 imported into the chloroplast in the absence of synthetic peptides was defined as 100%. Data shown in the figures are the means±s.d. of three independent experiments. TpL18, transit peptide added to L18; TpT14, transit peptide added to T14; input,in vitro-translated, radiolabeled precursors before the import reactions. (c) Effects of amino-acid substitution in the T14 region on pLHCP protein import.In vitroimport assays were performed for 5, 10, 15 and 20 min in the presence of pLHCP or amino-acid substitution mutants of pLHCP using chloroplasts isolated from 3-week-old seedlings. After import, intact chloroplasts were reisolated and analysed by SDS–PAGE. The gels were stained with Coomassie blue, scanned and dried for autoradiography. (d) Trypsin treatment after chloroplast protein import.In vitroimport assays were performed for 20 min in the presence of pLHCP or amino-acid substitution mutants of pLHCP using chloroplasts isolated from 3-week-old seedlings. After the import reaction, samples were incubated with 200 μg ml−1trypsin for 30 min on ice, chloroplasts were reisolated, and the proteins were separated by 15% SDS–PAGE and visualized by autoradiography. As shown in Figure 7a , pLHCP protein translocation was not affected by increasing concentrations of TpL18; however, pLHCP translocation was severely inhibited in the presence of the TpT14 in a concentration-dependent manner. The specificity of this inhibition was supported by the observation that TpT14 had no significant effect on the import of Sec pathway substrate pOE33 or Tat pathway substrate pOE23 ( Fig. 7b ). Figure 7: T14 is important for pLHCP protein translocation across the inner membrane. ( a ) A synthetic peptide corresponding to T14 competes with pLHCP for translocation across the envelope. Chloroplasts were isolated from 3-week-old Arabidopsis plants and incubated with [ 35 S]pLHCP, [ 35 S]pOE33 or [ 35 S]pOE23 for 10 min in the presence of increasing concentrations of TPT14 or TPL18 peptide (as described in the Methods). After incubation, the intact chloroplasts were reisolated, and the chloroplast proteins were separated on 15% SDS–PAGE gels and visualized by autoradiography. ( b ) Quantification of imported mature [ 35 S]LHCP, [ 35 S]OE33 or [ 35 S]OE23 relative to the amount of endogenous LHCP resolved by SDS–PAGE. The amount of mature [ 35 S]LHCP, [ 35 S]OE33 or [ 35 S]OE23 imported into the chloroplast in the absence of synthetic peptides was defined as 100%. Data shown in the figures are the means±s.d. of three independent experiments. TpL18, transit peptide added to L18; TpT14, transit peptide added to T14; input, in vitro -translated, radiolabeled precursors before the import reactions. ( c ) Effects of amino-acid substitution in the T14 region on pLHCP protein import. In vitro import assays were performed for 5, 10, 15 and 20 min in the presence of pLHCP or amino-acid substitution mutants of pLHCP using chloroplasts isolated from 3-week-old seedlings. After import, intact chloroplasts were reisolated and analysed by SDS–PAGE. The gels were stained with Coomassie blue, scanned and dried for autoradiography. ( d ) Trypsin treatment after chloroplast protein import. In vitro import assays were performed for 20 min in the presence of pLHCP or amino-acid substitution mutants of pLHCP using chloroplasts isolated from 3-week-old seedlings. After the import reaction, samples were incubated with 200 μg ml −1 trypsin for 30 min on ice, chloroplasts were reisolated, and the proteins were separated by 15% SDS–PAGE and visualized by autoradiography. Full size image Because the above results suggest that T14 is essential for pLHCP translocation across the envelope, we performed import reactions with pLHCP-DPLG, pLHCP-ELK and pLHCP-RLAM mutants to further test this possibility ( Fig. 7c ). There were no apparent changes in protein import between the pLHCP and Ala substitution pLHCP-DPLG. However, import of pLHCP-ELK and pLHCP-RLAM into the chloroplast stroma was greatly inhibited, with remarkably reduced amounts of mature proteins and increased levels of pLHCP. In addition, treatment of the chloroplasts with trypsin after the import reaction showed that mLHCP was protected from protease degradation ( Fig. 7d ). Nuclear-encoded chloroplast proteins are inserted into or translocated across the thylakoid membrane by four protein translocation pathways after import into the chloroplast [3] , [4] . We have attempted to uncover the molecular events that are responsible for routing imported proteins into these distinct pathways. In this study, we report the identification and functional characterization of the LTD protein, which is essential for the import of pLHCP and subsequent routing of these proteins to the cpSRP pathway. This study provides the first insight into the routing mechanisms of LHCP to cpSRP-dependent transport pathway within chloroplasts. The ltd mutant of Arabidopsis displays a severe pigment deficiency phenotype ( Fig. 1 ). Inactivation of LTD caused a severe decrease in the levels of various LHCPs and a mild decrease in the levels of photosynthetic protein complexes, but there was no effect on the accumulation of protein import components ( Fig. 1 and Supplementary Figure S3 ). As LHCII has been suggested to be involved in the assembly of thylakoid membranes into grana stacks [26] , the dramatic decrease in LHCP in ltd may cause the observed defect in thylakoid membrane structure. Previous studies demonstrated that several Arabidopsis mutants lacking cpSRP54, cpSRP43, cpSRP43/cpSRP54, cpFtsY and Alb3 showed different degrees of pigment deficiency phenotypes [16] , [21] , [23] , [28] , [29] , [34] . The ltd mutant did not develop any fertile flowers ( Fig. 1a ), indicating that LTD, similarly to cpFtsY and Alb3, is required for photoautotropic growth [21] , [34] , [35] . The presence of LTD at the envelope suggests that it possibly assists in pLHCP translocation across the envelope. Consistent with this hypothesis, LTD interacts with both precursor and mature LHCP ( Fig. 5a ). Previous studies have shown that the C-terminal region, including the third transmembrane domain of LHCP, was essential for the translocation of pLHCP into the chloroplast [39] , [40] . However, another report showed that its C terminus is not required for pLHCP import into the chloroplast [41] . The reason for this discrepancy is unclear. In this study we identified a T14 region (amino acids 211–224) at the beginning of the third LHCP transmembrane domain functioning as an LTD-binding segment that facilitates pLHCP translocation across the inner membrane, which agrees with the report on the function of its C terminus in protein import [39] , [40] . Several lines of evidence lend support for the function of T14 region in pLHCP import. First, a 5 amino-acid deletion in the T14 region of LHCP leads to the loss of interaction with LTD ( Fig. 6 ). Second, substitutions of several conserved amino acids in T14 severely affect pLHCP translocation efficiency ( Fig. 7 ). Third, synthetic peptides corresponding to TpT14 severely inhibited pLHCP translocation across the envelope but not the import of Sec- and Tat-dependent substrates. Meanwhile, the addition of TpL18 only slightly inhibited the translocation of pLHCP into the chloroplast ( Fig. 7 ). The interactions of LTD with Tic110 and Tic40 suggest that LTD function at the envelope is mediated through the interaction with TIC proteins. Tic110 and Tic40 have been proposed to have roles in the recruitment of stromal molecular chaperones to the stromal face of TIC [2] , [6] , [11] . The tic110 and tic40 mutant plants also showed dramatically reduced levels of LHCP, and had few granal stacks [8] , [42] , [43] . Thus, LTD may be specifically recruited to the envelope for pLHCP recognition and translocation across the inner membrane as they emerge from the TIC channel. Studies on the import and integration of LHCP into the thylakoid membrane have revealed that pLHCP is rapidly processed to its mature form on import, concomitantly with the formation of a soluble stromal transit complex, which is competent to be inserted into the membrane [22] , [44] . Interaction of LTD with newly imported LHCP during chloroplast import ( Fig. 5 ) suggests that LTD is likely to recruit the protease for the processing. LTD interacts with cpSRP43 but not with cpSRP54 and cpFtsY; however, the interaction between LTD and cpSRP43 is relatively weak ( Fig. 3 ). Thus, LTD may not form a stable complex with cpSRP43, which is consistent with the observation that LTD does not co-migrate with cpSRP43 and cpSRP54 ( Supplementary Fig. S4 ). LTD formed an intermediate complex with pLHCP, but a LTD–cpSRP43–pLHCP triple complex was not observed ( Fig. 5 ). In addition, a cpSRP43/cpSRP54/pLHCP transit complex was formed concomitantly with the disappearance of LTD–pLHCP complex when pLHCP was incubated with cpSRP43, cpSRP54 and LTD. Moreover, time course import experiments provide further support that LHCP first contacts LTD and is then handed over to cpSRP ( Fig. 5 ). cpSRP43 was found to be associated with mLHCP, but not pLHCP in chloroplast protein import assay ( Fig. 5a ); however, cpSRP43 efficiently forms a complex with pLHCP in vitro ( Fig. 5b ). In vitro reconstitution assay also showed that both precursor and mature LHCP can integrate into the thylakoid membrane [44] . The interaction of cpSRP43 with mLHCP may reflect the process after import into the chloroplast. Thus, these results suggest that LTD routes LHCP to the cpSRP pathway during or shortly after translocation across the inner envelope membrane into the stroma. The LTD protein contains ankyrin-repeat-containing domain, which has been implicated in mediating protein–protein interactions [45] . Several Arabidopsis ankyrin proteins have been shown to interact with substrate proteins and participate in the protein translocation process [16] , [46] . cpSRP43 contains a chromodomain at the N terminus, which is followed by four ankyrin repeats and then two chromodomains [16] . The ankyrin domain of cpSRP43 provides the binding site for the L18 region of LHCP and is involved in post-translational targeting of LHCP to the thylakoid membrane [18] , [36] . Another ankyrin protein, AKR2A, has been also shown to interact with the outer envelope membrane protein OEP7 and targets it to the chloroplast [46] . However, it is surprising that LTD specifically interacts with at least four different components (cpSRP43, LHCP, Tic40 and Tic110) given that LTD is rather small and has only one predicted ankyrin repeat. Previous results have also revealed several interaction partners of small proteins. Tim12, a small peripheral membrane subunit of TIM22 translocation component with a molecular mass of 12 kDa, has been shown to interact directly with Tim9, Tim10, Tim22 and carrier proteins, and delivers these carrier proteins to the inner membrane [47] , [48] . Distinct properties of N- and C-terminal ends of Tim12 have been demonstrated to be important for its interactions and functions [47] . It is likely that the LTD function may also rely on the distinct functional regions of this protein. The identification of LTD in LHCP import and subsequent delivery to the cpSRP pathway was unexpected, as both the envelope and cpSRP transport pathways have been extensively investigated and this component has not been detected before [11] , [15] , [20] , [21] , [49] , [50] . One possibility is that the inability of LTD to form the stable complexes with cpSRP43 or with Tic40 and Tic110, making it difficult to be detected using the biochemical assays currently applied in the identification of the components of the envelope and cpSRP transport pathways [11] , [15] , [20] , [21] , [49] , [50] . Another possibility is that an intermediate stage of such process cannot be trapped or reconstituted in vitro for further identification of the components involved in because the transport from the inner envelop to the SRP pathway is so rapid. Moreover, LTD cannot be identified by analogue with protein export pathway in mammalian and Escherichia coli . Homologues of prokaryotic SRP54 and its receptor FtsY have been identified in chloroplasts [15] , [20] . However, LTD and cpSRP43 homologues are found in higher plants, moss and green algae but not in cyanobacteria and red algae [23] ( Supplementary Fig. S1 ). It is possible that LTD and cpSRP43 are evolved after the origin of chloroplasts by endosymbiosis for LHCP biogenesis. Furthermore, the lack of extensive characterization of ltd and thorough studies of the LTD function may also account for this. Thus, in this study, we have taken genetic and biochemical approaches to uncover the unexpected, novel function of the LTD protein. The LTD protein was first suggested to be involved in the biogenesis of LHCP through biochemical analysis of the ltd mutant ( Fig. 1 ). Further subcellular localization studies ( Fig. 2 ) indicate that LTD likely functions in the early stages of LHCP translocation during or after import into the chloroplast. The interactions of LTD with TIC, cpSRP and LHCP, and its functions in LHCP targeting and sorting processes provide further evidence for the functions of LTD in facilitating the import of LHCP and subsequent routing of these proteins to the cpSRP pathway. These functions may be important for maintaining efficient targeting and sorting processes as well as preventing mistargeting to other pathways. It is possible that similar components may also exist for routing of imported proteins to other translocation pathways besides the cpSRP pathway. In summary, we propose a model based on the results described here ( Fig. 8 ): LTD is recruited to the envelope and recognizes the T14 region at the beginning of the third transmembrane domain of LHCP as LHCP emerge from the inner envelope translocation channel; then it directs the imported LHCP to the cpSRP pathway, in which cpSRP43 interacts with the L18 region between the second and third transmembrane domains of LHCP to form a transit complex with cpSRP54, resulting in targeting of LHCP to the thylakoid membrane. 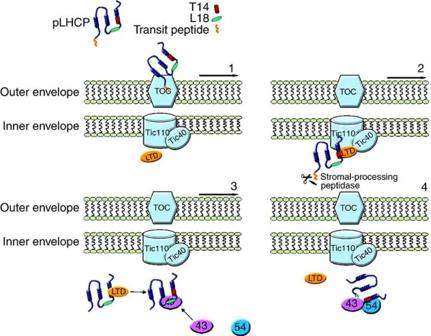Figure 8: A proposed model for LTD-mediated LHCP delivery to the cpSRP pathway. Nuclear-encoded pLHCP proteins are synthesized in the cytosol and post-translationally translocated across the chloroplast outer envelopes by the TOC complex (translocon at the outer envelop membrane of chloroplasts) and TIC complex (translocon at the inner envelop membrane of chloroplasts). During translocation across the TIC channel, LTD is recruited to the envelope and recognizes T14 at the beginning of the third transmembrane domain of LHCP as they emerge from the envelope translocation channel. At this stage, it is likely the stromal processing peptidase is also recruited for cleavage of the transit peptide. Then, LTD transiently interacts with cpSRP43 and delivers LHCP to the cpSRP pathway, in which cpSRP43 interacts with L18 between the second and third transmembrane domains and forms a transit complex with cpSRP54. Figure 8: A proposed model for LTD-mediated LHCP delivery to the cpSRP pathway. Nuclear-encoded pLHCP proteins are synthesized in the cytosol and post-translationally translocated across the chloroplast outer envelopes by the TOC complex (translocon at the outer envelop membrane of chloroplasts) and TIC complex (translocon at the inner envelop membrane of chloroplasts). During translocation across the TIC channel, LTD is recruited to the envelope and recognizes T14 at the beginning of the third transmembrane domain of LHCP as they emerge from the envelope translocation channel. At this stage, it is likely the stromal processing peptidase is also recruited for cleavage of the transit peptide. Then, LTD transiently interacts with cpSRP43 and delivers LHCP to the cpSRP pathway, in which cpSRP43 interacts with L18 between the second and third transmembrane domains and forms a transit complex with cpSRP54. Full size image Isolation and growth conditions of the ltd mutant The T-DNA insertion lines ltd (SALK_126967C), cpftsY (SALK_049077) [34] and ffc mutant (CS850421) were obtained from the Arabidopsis Biological Resources Centers, and the homozygous mutants and precise T-DNA insertion sites were confirmed by PCR and sequencing with primers A, C and LB1 (all primer sequences are listed in Supplementary Table S1 ) for ltd ; primers LP54, RP54 and LB2 for ffc ; and primers FtsYF, FtsYR and LB1 for cpftsY . The chaos mutant and chaos/ffc double mutant were kindly provided by Dr Laurent Nussaume [23] , [29] . Wild-type and homozygous mutant plants were grown on Murashige and Skoog (MS) media supplemented with 3% sucrose under short-day conditions (10 h of light/14 h of dark) with a photon flux density of 80 μmol m −2 s −1 in a growth chamber at 22 °C. For complementation of the ltd phenotype, a fragment containing the full-length LTD- coding sequence was amplified with the primers LTDcomF and LTDcomR. The PCR product was digested with Kpn I and Sac I and subcloned into the pSN1301 vector under the control of the cauliflower mosaic virus 35S promoter. The construct was transferred to heterozygous LTD plants by Agrobacterium tumefaciens -mediated transformation using the floral dip method [51] . Transgenic plants were selected on MS medium containing 50 mg l −1 hygromycin and grown in a greenhouse to produce seeds for PCR analysis. The success of complementation was confirmed by immunoblot analysis. The expression of LTD ( At1g50900 ) was determined by reverse transcription–PCR using the primers LTDRTF and LTDRTR. To ensure equal amounts of RNA were used for each sample, reverse transcription–PCR analysis of the actin cDNA was performed using the actinF and actinR primers. Total protein preparation and immunoblot analysis Total proteins were extracted from Arabidopsis leaves [52] and from yeast strain NMY32 (ref. 53 ). Protein concentrations were determined using the Bio-Rad DC protein assay (Bio-Rad). For immunoblot analysis, total proteins were separated by SDS–PAGE and transferred to nitrocellulose membranes. The membranes were incubated with specific primary antibodies, and signals from secondary conjugated antibodies were detected by enhanced chemiluminescence. Yeast two-hybrid assays Gal4-based yeast two-hybrid assays were performed using the Matchmaker Gold Yeast Two-Hybrid System from Clontech according to the manufacturer's instructions. The vectors pGADT7 and pGBKT7 were used to construct the prey and bait plasmids, respectively. The plasmids constructed for yeast assays are listed in Supplementary Table S1 . Y2HGold yeast cells containing each of the activation domain constructs were transformed with each of the binding domain constructs and plated on synthetic dropout (SD) medium containing 10 μg l −1 X-α-Gal (5-bromo-4-chloro-3-indolyl-α- D -galactopyranoside) without tryptophan, leucine and histidine. β-Galactosidase activity was assayed in the presence of X-α-Gal. Split ubiquitin-based yeast two-hybrid assays were performed using the yeast strain NMY32 supplied by Dualsystems Biotech [54] . The pCCW vector encoding the Cub-LexA-VP16 fragment was used to construct the bait plasmids. The prey plasmids were constructed from the vector pDSLNx, which encodes the NubG fragment (Dualsystems Biotech). Plasmids constructed for the yeast assays are listed in Supplementary Table S1 . Interactions were determined by growing diploid yeast colonies on SD-His-Leu-Trp plates and by β-galactosidase activity using an X-gal (5-bromo-4-chloro-3-indolyl-b- D -galactopyranoside) filter assay. NMY32 containing x-Cub-LexAVP16 (x represents various deletion mutants of LHCP) was transformed with the NubI-Alg5 expression plasmid as a positive control, and NMY32 containing x-Cub-LexA-VP16 was transformed with the plasmid expressing NubG-Alg5 as a negative control. In vitro translation of precursor proteins and protein import Fragments encoding full-length Lhcb1, OE23 and OE33 were amplified using the following primers: Lhcb1TNTF and Lhcb1TNTR for pLHCP; OE23TNTF and OE23TNTR for pOE23; and OE33TNTF and OE33TNTR for pOE23 ( Supplementary Table S1 ). Amplified PCR products were cleaved and subcloned into the EcoRI-SalI sites of the pTNT expression vector (Promega). Transcription/translation was performed using a wheat germ system (Promega) containing [ 35 S]-methionine and SP6 RNA polymerase according to the manufacturer's instructions. The pLHCP substitution mutants were generated using the Fast mutagenesis system (Trans Gen Biotech). Chloroplast isolation and protein import assays were performed as described previously [55] with the following modifications. Briefly, 3-week-old Arabidopsis plants were homogenized in isolation buffer (0.33 M sorbitol, 5 mM MgCl 2 , 5 mM EGTA and 5 mM EDTA, 50 mM HEPES-KOH pH 8.0, and 10 mM NaHCO 3 ), filtered through Miracloth and centrifuged for 1 min at 1,000 g . The pellets were resuspended and loaded onto Percoll step gradients (40 and 70% in isolation buffer), and chloroplasts were collected and washed twice with import buffer (50 mM HEPES-KOH, pH 8.0, 3 mM MgSO 4 and 0.33 M sorbitol). For protein import, chloroplasts at a final concentration of 0.2 mg ml −1 chlorophyll were incubated with 8 μl precursor in 100 μl import buffer supplemented with up to 5 mM ATP. Import reactions were performed in white light (100 μmol m −2 s −1 ) at 25 °C. To examine the effects of the T14 and L18 peptides on protein import, TpL18 (transit peptide fused to the L18 peptide (MAASTMALSSPAFAGKAVNLSPADLLYPGGSFDPLGLATDP)) and TpT14 (transit peptide fused to the T14 peptide (MAASTMALSSPAFAGKAVNLSPAELKVKELKNGRLAM); >80% purity by Seajetsci) were added to the import reaction buffer, and import was performed for 10 min. For protease digestion of intact chloroplasts, the import reaction was incubated for 20 min and then was supplemented with 200 μg ml −1 trypsin for 30 min on ice, and trypsin reactions were quenched by addition of a protease inhibitor cocktail with final concentrations of 100 μg ml −1 phenylmethanesulfonyl fluoride, 1 μg ml −1 aprotinin, 1 μg ml −1 pepstatin and 1 μg ml −1 E64 (3-carboxy-trans-2,3-epoxypropyl-leucylamido-(4-guanidino)butane). Chloroplasts were collected through a 40% Percoll cushion at 4 °C, separated on 15% SDS–PAGE gels and analysed by autoradiography. Chloroplast fractionation and overlay analysis Intact chloroplasts were fractionated into the outer and inner envelope, stromal and thylakoid membrane fractions as described previously [56] . For the protein overlay assay, the fractionated stromal or inner envelope proteins were separated by SDS–PAGE and transferred to nitrocellulose membranes, which were blocked with TTBS buffer (20 mM Tris-HCl, pH 7.6, 0.137 M NaCl, and 0.1% Tween-20) containing 5% skimmed milk and incubated with the recombinant LTD or cpSRP43 proteins carrying a polyhistidine tag at both their N- and C-terminus at a concentration of 0.1 mg ml −1 in TTBS buffer with 1% skimmed milk. The membrane was washed three times with TTBS buffer, probed with an anti-His-tag antibody and visualized by the enhanced chemiluminescence method. Pull-down and co-immunoprecipitation assays Fifty-microliter aliquots of 50% glutathione-agarose beads were washed with buffer (10 mM Tris-HCl, pH 7.5, 1 mM EDTA, 1 mM EGTA, 0.5% NP40, 1% Triton X-100, 150 mM NaCl and 1 mM DTT) three times, then 4 μg purified bait and 4 μg pre-cleared prey proteins were added to a final volume of 100 μl. After incubation in 10 mM Tris-HCl, pH 7.5, 1 mM EDTA, 1 mM EGTA, 0.5% NP40, 1% Triton X-100, 150 mM NaCl and 1 mM DTT for 4 h at 4 °C, unbound proteins were removed by washing for three times. The bound proteins were eluted and separated by SDS–PAGE followed by immunoblot analysis or Coomassie staining. To analyse the interactions of LTD with import precursors, in vitro -translated [ 35 S]pLHCP was incubated with isolated Arabidopsis chloroplasts under white light (100 μmol m −2 s −1 ) at 25 °C with 1 mM ATP for 5 min, and chloroplasts were collected through a 40% Percoll cushion at 4 °C. The pellets were solubilized with 1% docecyl β- D maltoside in the presence of 50 mM HEPES-KOH, pH 8.0, 150 mM NaCl and 4 mM MgCl 2 , and the supernatant was collected by centrifugation at 180,000 g for 45 min. For immunoprecipitation, antibodies were added to the clarified supernatant, which was incubated overnight at 4 °C and then precipitated with Protein-A-agarose. After washing the beads with 50 mM HEPES-KOH, pH 8.0, 150 mM NaCl and 4 mM MgCl 2 five times, the bound proteins were eluted, separated on 15% SDS–PAGE gels and analysed by immunoblot and autoradiography. Subcellular localization of GFP proteins DNA encoding the full-length LTD protein was amplified by PCR using prime LTDGFPF and prime LTDGFPR, and the PCR products were ligated into the GFP fusion vector pUC18-35s-sGFP with GFP as a reporter. The constructs for nuclear, chloroplast and mitochondria localization were constructed according to the previous methods [31] , [32] , [33] . The resulting fusion constructs and the control vector were introduced into wild-type Arabidopsis . The GFP in the examined samples was performed as described previously [31] . In vitro reconstitution analysis [ 35 S]pLHCP, which was synthesized in wheat germ extracts according to the method described above, was mixed with recombinant LTD (200 ng), cpSRP43 (400 ng) or cpSRP54 (200 ng) in import buffer in the presence of 1 mM ATP in a final volume of 50 μl for 15 min at 25 °C. All samples contained equal amounts of wheat germ extract. The samples were separated on 6–12% nondenaturing polyacrylamide gels [57] , and the resolved protein complexes were visualized by autoradiography. Transmission electron microscopy Samples of 3-week-old wild-type and mutant leaves were fixed as described in Peng et al . [58] Micrographs were taken using a transmission electron microscope (JEM-1230; JEOL). How to cite this article: Ouyang, M. et al . LTD is a protein required for sorting light-harvesting chlorophyll-binding proteins to the chloroplast SRP pathway. Nat. Commun. 2:277 doi: 10.1038/ncomms1278 (2011).